Changes in the regulation of cortical neurogenesis contribute to encephalization during amniote brain evolution The emergence of larger brains with large numbers of neurons is an evolutionary innovation in mammals and birds. However, the corresponding changes in cortical developmental programmes during amniote evolution are poorly understood. Here we examine the cortical development of Madagascar ground geckos, and report unique characteristics of their reptilian cortical progenitors. The rates of proliferation and neuronal differentiation in the gecko cortex are much lower than those in other amniotes. Notch signalling is highly activated in the gecko cortical progenitors, which provides a molecular basis for the low rate of cortical neurogenesis. Interestingly, multiple neuron subtypes are sequentially generated in the gecko cortex, similar to other amniotes. These results suggest that changes in the regulation of cortical neural progenitors have accelerated neurogenesis and provided encephalization in mammalian and archosaurian lineages. In addition, the temporal regulation for making cortical neuronal subtypes has evolved in a common ancestor(s) of amniotes. There is great diversity in the size and complexity of organs among animals, which reflects the diverse physiological capabilities necessary to adapt to various ecological niches [1] . Variations in organ morphology are primarily dependent on differential growth rates during the embryonic and post-embryonic periods [2] . Several developmental parameters, such as the duration of organogenesis and the relative abundance of cell proliferation, differentiation and cell death, vary among species and are critical to create the species-specific architectures of organs [3] , [4] , [5] . For centuries, evolutionary changes in vertebrate brain morphology have been of particular interest to neuroscientists [6] , [7] . Brain-body scaling indicates that mammals and birds have relatively large brains compared with other vertebrate species [8] . Furthermore, the dorsal region of the telencephalon (pallium) in these animals is elaborated in distinct ways. The mammalian pallium gives rise to the neocortex, a conspicuous structure characterized by the tangential expansion of the surface area and a six-layered lamination [9] . In contrast, the avian dorsal pallium gives rise to the Wulst or hyperpallium, which is not composed of tangential laminar sheets, but rather of nuclear structures with similar neuronal characteristics [10] . These anatomical hallmarks are constructed with large numbers of neurons of a variety of subtypes, which are generated by the rapid expansion of neural stem/progenitor cells in the early embryonic stages followed by the sequential production and migration of distinct neuronal subtypes during embryogenesis [11] . Recent studies have shown that the differential regulations of neuronal subtype specification and migration underlies the formation of mammalian- and avian-specific pallial structures [12] , [13] , [14] . However, the regulatory mechanisms underlying the increased size of the pallium and the evolutionary origin of multiple subtypes of pallial neurons remain to be elucidated. As all extant amniotes have diverged from ancestral groups of reptiles [15] , modern reptiles, including lepidosaurs and non-avian archosaurs ( Fig. 1a ), may possess plesiomorphic traits inherited from the common ancestor of amniotes. Indeed, compared with mammals and birds, the extant reptiles have relatively small brains, and their cortex consists of a three-layered laminar structure [16] . These characteristics of the reptilian brain were thought to be an evolutionary intermediate between amphibian and mammalian/avian brains [17] , [18] . However, cellular and molecular analyses of reptilian cortical development have been extremely limited owing to technical difficulties in embryonic manipulation. 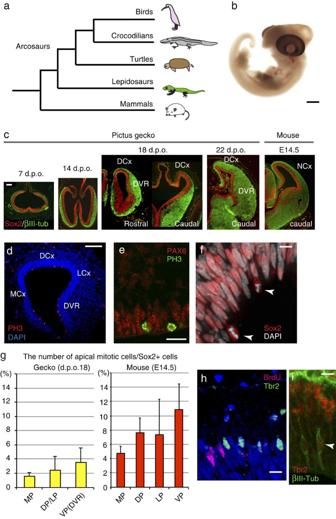Figure 1: Cortical development in geckos. (a) A phylogenic tree of amniotes. The position of the turtles is based on a recent report46,47. (b) An gecko embryo (P. pictus; 18 d.p.o.). (c) The ontogeny of the telencephalon in the gecko (left, from 7 to 22 d.p.o.) is shown alongside a comparable stage of telencephalon development in the mouse (right, E14.5). Immunostaining was performed with anti-Sox2 and anti-ß III tubulin antibodies. (d–f) The distribution of mitotic cells in the developing gecko ventricular zone. Phosphorylated histone H3-positive mitotic cells are scattered on the apical side of the ventricular zone that is distinguished by PAX6 (e) and Sox2 (f) expression. (g) The proportion of mitotic cells in the gecko cortex (18 d.p.o.; left graph) compared with that in the mouse cortex (E14.5; right graph). Values represent mean (n=3 animals) and s.d. (h) The distribution of Tbr2-positive cells and BrdU-labelled cells in the ventricular zone of the developing gecko cortex. (i) Co-expression of Tbr2 and ß III tubulin (an arrowhead). Scale bars, 200 μm (c), 50 μm (d) and 20 μm (f,h,i). Figure 1: Cortical development in geckos. ( a ) A phylogenic tree of amniotes. The position of the turtles is based on a recent report [46] , [47] . ( b ) An gecko embryo ( P. pictus ; 18 d.p.o.). ( c ) The ontogeny of the telencephalon in the gecko (left, from 7 to 22 d.p.o.) is shown alongside a comparable stage of telencephalon development in the mouse (right, E14.5). Immunostaining was performed with anti-Sox2 and anti-ß III tubulin antibodies. ( d – f ) The distribution of mitotic cells in the developing gecko ventricular zone. Phosphorylated histone H3-positive mitotic cells are scattered on the apical side of the ventricular zone that is distinguished by PAX6 ( e ) and Sox2 ( f ) expression. ( g ) The proportion of mitotic cells in the gecko cortex (18 d.p.o. ; left graph) compared with that in the mouse cortex (E14.5; right graph). Values represent mean ( n =3 animals) and s.d. ( h ) The distribution of Tbr2-positive cells and BrdU-labelled cells in the ventricular zone of the developing gecko cortex. ( i ) Co-expression of Tbr2 and ß III tubulin (an arrowhead). Scale bars, 200 μm ( c ), 50 μm ( d ) and 20 μm ( f , h , i ). Full size image Here, we focus on the Madagascar ground gecko ( Paroedura pictus ), a species of geckonoids, which are included in lepidosaurs ( Fig. 1b ). The Pictus gecko exhibits several unique characteristics, such as high reproductive activity in all seasons and a hard-shelled egg, which are highly advantageous for experimental biology [19] . We establish embryonic manipulation of the gecko and determine that the neural stem/progenitor cells in the developing gecko cortex have a low neurogenic potential. Canonical Notch signalling, which constrains the neurogenic potential of neural stem/progenitor cells, is highly activated in the gecko cortical ventricular zone, compared with other amniotes. Interestingly, the sequential generation of lamina-specific neuronal subtypes is evident in the gecko cortex, as is the case in mammalian and avian pallial development. These results suggest that changes in the rate of neurogenesis have occurred independently in mammalian and archosaurian lineages, and have resulted in the convergent encephalization that occurred during amniote brain evolution. In contrast, the temporal regulation of neuronal subtype specification is a shared feature of various amniote species, which implies that this trait is inherited from a common ancestor of amniotes. Lower proliferative activity in the developing gecko cortex To address reptilian cortical neurogenesis, we first examined the ontogeny of the cortical development in the Madagascar ground geckos. Neural stem/progenitor cells and differentiated neurons in the gecko cortex were distinguished by their expression of Sox2 and ßIII-tubulin, respectively ( Fig. 1c ). At 7 days of post-oviposition (d.p.o. ), the first cortical neurons appeared at the surface of the telencephalic vesicles, just above the Sox2-positive ventricular zone. As embryogenesis proceeded, the volume of the telencephalon and the thickness of the cortical neuronal layer were gradually increased, whereas the thickness of the cortical ventricular zone decreased proportionately ( Fig. 1c and Supplementary Fig. S1 ). The proportions of the ventricular zone and the neuronal layer in the gecko cortex at ~14–18 d.p.o. were comparable to those of the mouse cortex at embryonic days 12–14 ( Fig. 1c ). To determine the total neurogenic period in the gecko cortex, we administered 5-ethynyl-2′-deoxyuridine (EdU) into the gecko brain at various embryonic stages and analysed EdU-labelled cells in the dorsal cortex (DCx) at later stages. The number of EdU-positive cells was gradually decreased with progressing EdU administration stages, and none of the cortical neurons were labelled by the injection of EdU at 23 d.p.o. ( Supplementary Fig. S1 ). These results suggest that cortical neurogenesis terminates by 23 d.p.o. Thus, the total length of the cortical neurogenic period in the gecko is much shorter than the total length of embryogenesis (60–80 days between oviposition and hatching [19] ), similar to other reptilian species [20] , [21] ( Supplementary Table S1 ). The increase of cortical thickness at later embryonic stages in the gecko cortex was owing to massive elaboration of dendrites and axon bundles, rather than the increase of neuron numbers ( Supplementary Fig. S2 ). Next, we addressed the cell division in the developing gecko cortex. Immunostaining of phosphorylated histone H3 distinguishes M-phase cells during mitosis. At 14 d.p.o., which is the middle stage of corticogenesis, mitotic cells were scattered at the apical side of the gecko cortical ventricular zone ( Fig. 1d–f ). The frequency of mitotic cells exhibited a medial-low to lateral-high gradient, which is similar to the range in mouse ( Fig. 1g ) and chicken pallia [13] . Notably, the ratio of mitotic cells to Sox2-positive ventricular neural stem/progenitor cells was three times lower in the gecko cortex than in the mouse neocortex at E14.5 ( Fig. 1g ). Furthermore, we could not detect any mitotic features on the basal side of the ventricular zone, which suggests that the gecko cortex lacks subventricular basal progenitors ( Fig. 1d,e ). Interestingly, the expression of Tbr2, which delineates a subpopulation of basal progenitors in the mammalian neocortex [22] , was detected on the basal side of the gecko ventricular zone ( Fig. 1h ). In contrast to the mouse cortex, Tbr2-positive cells in the gecko cortex did not incorporate bromodeoxyuridine (BrdU) and were positive for ßIII-tubulin, indicating that these cells are post-mitotic neurons ( Fig. 1h,i ). These results indicate that the lower frequency of cell division at the apical ventricular side and the absence of basal progenitors are characteristics of the developing gecko cortex. Prolonged cell-cycle length in gecko corticogenesis The lower frequency of apical cell division in the gecko cortex might result from an extended cell-cycle length in cortical neural stem/progenitor cells. To determine the cell-cycle length in the proliferating cells of the gecko cortex, we used two-coloured pulse labelling in cycling cells ( Fig. 2a,b ). The administration of distinct thymidine analogues, EdU and BrdU, at different time points enabled us to determine the cell-cycle kinetics of proliferating cells [23] . The total number of proliferating cells was estimated by quantifying Sox2-positive cells in the ventricular zone. Two-coloured pulse labelling analysis indicated that the total length of the cell cycle (Tc) of neural stem/progenitor cells in the gecko DCx at 18 d.p.o. was 50.9±6.0 h ( Fig. 2c ), which was remarkably longer than that that of neural stem/progenitors in the developing mouse cortex (Tc=8–18 h [24] ). However, the length of S phase (Ts) in the gecko cortex was 5.4±1.3 h, which is comparable to that in the mouse cortex (Ts=3–5 h). This similarity suggests that S-phase duration is constant in amniotes and that the longer cell cycle in the gecko results from a lengthening of other cell-cycle phases such as G1 phase. Similar cell-cycle kinetics were obtained from the proliferating cells at the lateral part of the telencephalon, which gives rise to the dorsal ventricular ridge ( Fig. 2c ), indicating that long cell-cycle duration is common in all regions of the gecko telencephalon. 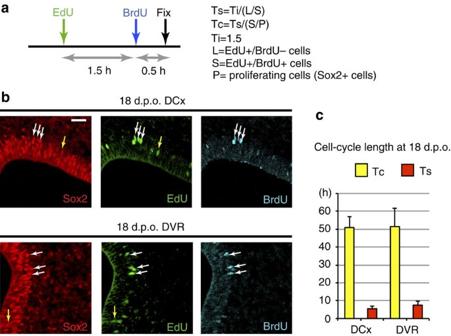Figure 2: Cell proliferation and cell-cycle length in the developing gecko cortex. (a) Calculation of cell-cycle length in the gecko ventricular zone. Sequential admnistration of EdU and BrdU estimates the total length of the cell cycle and S phase in neural stem/progenitors. (b) Immunostaining of the gecko DCx (upper panels) and dorsal ventricular ridge (DVR, lower panels) with anti-Sox2, EdU and BrdU antibodies. White arrows indicate Sox2+/EdU+/BrdU+ cells, and yellow arrows indicate Sox2+EdU+/BrdU− cells. (c) Quantifictaion of total cell-cycle length (Tc) and S phase (Ts) in the gecko DCx and DVR. Values represent mean (n=2 animals) and range. Scale bar, 100 μm. Figure 2: Cell proliferation and cell-cycle length in the developing gecko cortex. ( a ) Calculation of cell-cycle length in the gecko ventricular zone. Sequential admnistration of EdU and BrdU estimates the total length of the cell cycle and S phase in neural stem/progenitors. ( b ) Immunostaining of the gecko DCx (upper panels) and dorsal ventricular ridge (DVR, lower panels) with anti-Sox2, EdU and BrdU antibodies. White arrows indicate Sox2+/EdU+/BrdU+ cells, and yellow arrows indicate Sox2+EdU+/BrdU− cells. ( c ) Quantifictaion of total cell-cycle length (Tc) and S phase (Ts) in the gecko DCx and DVR. Values represent mean ( n =2 animals) and range. Scale bar, 100 μm. Full size image A low proportion of neuron-generating division in geckoes To visualize neural stem/progenitor cell behaviours of the developing gecko cortex, we performed in vivo electroporation into the developing gecko cortex, and traced the morphology and dynamics of ventricular cells using a green fluorescent protein (GFP) expression vector ( Fig. 3a,b ). Two days after electroporation, GFP expression was detected in Sox2-positive ventricular cells with long and direct radial fibres extending towards the surface of the cortex ( Fig. 3c ). Four days after electroporation, a subset of GFP-labelled cells began to express Tbr2 on the basal side of the ventricular zone. Some GFP-positive cells left the ventricular zone and extended multiple processes that were positive for ßIII-tubulin, which indicates that these were differentiated neurons ( Fig. 3d ). 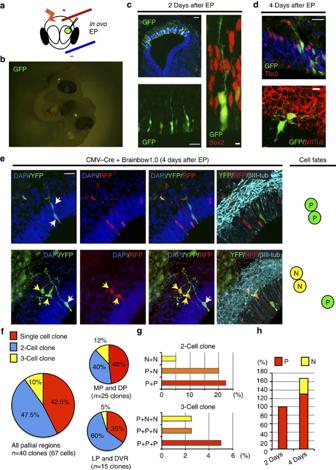Figure 3: Clonal analysis of neural stem/progenitor cells in the developing gecko cortex. (a–d) Electroporation of the GFP expression vector into the developing gecko cortex. (a) A schematic of electroporation. (b) A whole-mount view of gecko embryos electroporated with the GFP expression vector at 14 d.p.o. (c,d) The characteristics of GFP-expressing cells in the gecko cortex at 2 days (c) and 4 days (d) after electroporation. (e–h) Clonal analysis of the gecko cortex using the Brainbow system. (e) Recombined clones of gecko neural stem/progenitor cells at 4 days after electroporation. The upper panels show two pairs of clonal progenitors (white arrows). The lower panels show different clones including two pairs of neurons (yellow arrows) and a single progenitor (white arrow). (f) The proportion of single-cell, two-cell and three-cell clones at 4 days after electroporation. (g) Expansion of recombined progenitors and neurons from 2 days to 4 days after electroporation. (h) The identities of sibling cells in two-cell and three-cell clones at 4 days after electroporation. Scale bars, 100 μm (c, left upper panel), 50 μm (c, left lower panel;d, upper panel;e) and 10 μm (c, right panel;d, lower panel). Figure 3: Clonal analysis of neural stem/progenitor cells in the developing gecko cortex. ( a – d ) Electroporation of the GFP expression vector into the developing gecko cortex. ( a ) A schematic of electroporation. ( b ) A whole-mount view of gecko embryos electroporated with the GFP expression vector at 14 d.p.o. ( c , d ) The characteristics of GFP-expressing cells in the gecko cortex at 2 days ( c ) and 4 days ( d ) after electroporation. ( e – h ) Clonal analysis of the gecko cortex using the Brainbow system. ( e ) Recombined clones of gecko neural stem/progenitor cells at 4 days after electroporation. The upper panels show two pairs of clonal progenitors (white arrows). The lower panels show different clones including two pairs of neurons (yellow arrows) and a single progenitor (white arrow). ( f ) The proportion of single-cell, two-cell and three-cell clones at 4 days after electroporation. ( g ) Expansion of recombined progenitors and neurons from 2 days to 4 days after electroporation. ( h ) The identities of sibling cells in two-cell and three-cell clones at 4 days after electroporation. Scale bars, 100 μm ( c , left upper panel), 50 μm ( c , left lower panel; d , upper panel; e ) and 10 μm ( c , right panel; d , lower panel). Full size image During mammalian corticogenesis, symmetric progenitor–progenitor division increases the progenitor pool, whereas asymmetric neuron-producing division generates vast numbers of cortical neurons [25] . To address the frequency and the type of cell divisions occurring at middle stages of gecko corticogenesis, we conducted an in vivo clonal analysis of cortical neural stem/progenitor cells with a conditional multi-colour reporter system. We used the Brainbow1.0L vector, which expresses distinct colours of fluorescent proteins (RFP, YFP and CFP) following Cre-mediated recombination [26] . Electroporation of the Brainbow vector together with a Cre expression vector at a low concentration (1 ng μl −1 ) induced recombination at a clonal density [27] . Different recombination frequencies for multiple copies of the vectors provided different colour combinations in each clone ( Supplementary Fig. S3 ); however, we could not detect CFP-positive clones, most likely owing to preferential recombination of specific loxP sequences [28] . Importantly, the expression levels of the fluorescent proteins were maintained even after several rounds of cell divisions, confirming that the plasmid-based Brainbow system can be utilized for clonal analysis at least for a short period during development ( Supplementary Fig. S3 ). After electroporation of the gecko cortex, we quantified the number of cells in each recombined clone and determined the identity of the daughter cells as progenitors (P) or neurons (N) according to their morphology (radial glial or multipolar neuronal), position (the ventricular or the mantle zone) and marker expression (ßIII-tubulin) ( Fig. 3e ). At 2 days after electroporation, we confirmed that all of the recombined cells were single progenitor cells ( Supplementary Fig. S3 ). Surprisingly, even 4 days after electroporation, large numbers of recombinants still remained as single progenitor cells, indicating that these cells did not undergo cell division after recombination (42.5% of recombinants, n =40 clones, Fig. 3f ). The number of two-cell clone was slightly higher in the lateral/ventral pallium than in the medial/dorsal pallium, which is consistent with the medial-low to lateral-high gradient of proliferation activity in the gecko cortex. Among two-cell clones, P+P and P+N clones were observed in similar proportions ( Fig. 3g ), indicating that symmetric and asymmetric divisions had occurred with equal frequencies. Interestingly, a small population N+N clones were also detected, which suggests that a few committed neuronal precursors exist in the gecko ventricular zone. These trends were similar in three-cell clones that comprise all possible combinations of daughter cells (P+P+P, P+P+N and P+N+N), although the majority were progenitor cell clones (P+P+P, Fig. 3g ). Using these data, we quantified the proportions of P and N cells among the recombined cells and estimated the rates of progenitor and neuron expansion after recombination ( Fig. 3h ). At 4 days after electroporation (18 d.p.o. ), the proportion of P cells was much greater than that of N cells (77.9% of P cells and 22.1% of N cells), indicating that the majority of clones that originated from single neural stem/progenitor cells predominantly contributed to the maintenance of the progenitor pool rather than the expansion of neurons. This conclusion is suggested primarily by the low frequency of cell division and the prevailing occurrence of symmetric P+P division rather than asymmetric neuron-generating division. These lines of evidence indicate that gecko neural stem/progenitor cells predominantly and slowly undergo self-renewing division, which results in a minimal generation of cortical neurons. Comparison of cortical neuronal outputs in amniotes To investigate differences in cortical neurogenic rates between species, we compared the frequencies of neuronal differentiation in the dorsal pallia of various amniotes, including mice, geckos, turtles (Chinese soft-shelled turtles; Pelodiscus sinensis ) and chickens. We labelled pallial neural stem/progenitor cells by administering EdU or electroporating a GFP expression vector, and examined the proportion of EdU- or GFP-labelled neurons. Neuronal output was examined at different embryonic stages during the cortical/pallial neurogenic period in each species [21] , [24] , [29] ( Fig. 4a ). In mouse and chicken embryos, a large number of EdU- or GFP-positive cells migrated from the ventricular zone and differentiated into neurons at just 1 day after pulse labelling (17–54% of total EdU- or GFP-labelled cells; Fig. 4b,c and Supplementary Fig. S4 ). The rapid and massive neuronal differentiation in the mouse and chicken embryos was evident in all stages examined. In contrast, the frequency of neuronal differentiation was increased slowly in gecko embryos, in which a large number of EdU- or GFP-positive cells still remained in the ventricular zone and expressed Sox2 at 2 days after pulse labelling ( Fig. 4b,c and Supplementary Fig. S4 ). Interestingly, the frequency of neuronal output was higher in turtles than in geckos: the percentage of neurons among GFP-positive cells at 2 days after pulse labelling was 25.6% in turtles (14 d.p.o.) and 1.5% in geckoes (14 d.p.o.). These results indicate that the proportion of neuronal output varies greatly among species, which is most likely because of the species-specific proliferation/differentiation kinetics of cortical neural stem/progenitor cells. The differences in the neurogenic frequency between geckos and turtles also imply that these reptilian species have distinct regulatory mechanisms for cortical neuronal differentiation. 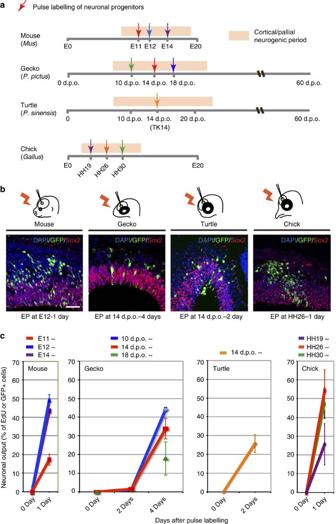Figure 4: Comparison of neurogenic rates in distinct amniote species. (a) A diagram showing the cortical/pallial neurogenic period in different amniotes, including mouse, gecko (P. pictus), turtle (P. sinensis, Chinese soft-shelled turtle) and chicken. Pulse labelling of neural stem/progenitor cells was performed by the administration of EdU or electroporation of GFP expression vectors. (b) Neuronal differentiation traced by the electroporation of the GFP expression vector in the developing cortices of the mouse, gecko and turtle, as well as in the chicken pallium. The ventricular zone is distinguished by Sox2 expression. (c) The proportion of EdU- or GFP-labelled differentiated neurons in the mouse, gecko and turtle cortices as well as in the chicken pallium after pulse labelling at various embryonic stages. Values represent mean (n=3 animals) and s.d. Scale bar, 100 μm. Figure 4: Comparison of neurogenic rates in distinct amniote species. ( a ) A diagram showing the cortical/pallial neurogenic period in different amniotes, including mouse, gecko ( P. pictus ), turtle ( P. sinensis , Chinese soft-shelled turtle) and chicken. Pulse labelling of neural stem/progenitor cells was performed by the administration of EdU or electroporation of GFP expression vectors. ( b ) Neuronal differentiation traced by the electroporation of the GFP expression vector in the developing cortices of the mouse, gecko and turtle, as well as in the chicken pallium. The ventricular zone is distinguished by Sox2 expression. ( c ) The proportion of EdU- or GFP-labelled differentiated neurons in the mouse, gecko and turtle cortices as well as in the chicken pallium after pulse labelling at various embryonic stages. Values represent mean ( n =3 animals) and s.d. Scale bar, 100 μm. Full size image Inter-species differences in Notch activation levels To identify the molecular mechanisms underlying inter-species differences in the rate of neuronal differentiation, we focused on Notch signalling, which has a crucial role in the maintenance of neural stem/progenitor cells in the embryonic brains. Upon activation, the intracellular domain of the Notch receptor (NICD) translocates to the nucleus and interacts with the transcription factor RBP-Jk (also known as CSL or CBF1), which regulates various downstream genes that are essential for maintaining stemness [30] . First, we addressed the expression of RBP-Jk in the cortical/pallial neural stem/progenitor cells of various amniote species. The expression of RBP-Jk was detected in neural stem/progenitor cells of developing mouse, gecko, turtle and chicken cortices/pallia ( Supplementary Fig. S5 ). Next, to examine the distribution of Notch signalling-activated cells in the developing cortex/pallium, we utilized a reporter vector containing CSL-responsive elements upstream of GFP, which faithfully reports RBP-Jk-dependent canonical Notch signalling [31] . The Notch reporter vector was electroporated into the dorsal telencephalon of mouse, gecko, turtle and chicken embryos ( Fig. 5 ). To trace electroporated cells, a vector that expresses mRFP under the control of the CMV promoter was co-electroporated with the reporter vector. Two days after electroporation, the expression of GFP (Notch reporter) was observed in Sox2-positive ventricular cells in all amniotes examined ( Fig. 5a ). However, there were significant inter-species differences in the proportion of Notch reporter-positive cells. In mice, only a subset of mRFP-positive ventricular cells highly expressed GFP (46.1±5.1% of total RFP/Sox2+ cells, n =3 animals, Fig. 5c ), whereas other cells exhibited low levels of GFP expression or were GFP-negative, as previously reported [32] . Mosaic patterns of GFP expression in neural stem/progenitor cells were also observed in the developing cortices/pallia of turtle and chicken embryos (36.6±2.4% of total RFP/Sox2+ cells in turtles, n =2 animals; 40.6±8.8% of total RFP/Sox2+ cells in chicken, n =3 animals; Fig. 5c ). In contrast, almost all of the mRFP-positive cells in the ventricular zone of the gecko cortex highly expressed GFP in the gecko cortex (97.2±3.95% of total RFP/Sox2+ cells, n =3 animals, Fig. 5c ). To quantify the activation level of Notch signalling among different species, we electroporated a 4 × CSL-luciferase vector into the mouse, gecko and chicken cortices/pallia at distinct embryonic stages and performed a luciferase reporter assay. In mouse and gecko cortices, the promoter activity of the Notch reporter vector was increased by the progression of embryonic stages; geckos exhibited higher levels of promoter activities than other species, particularly at later embryonic stages ( Fig. 5c ). Interestingly, the promoter activity of Notch reporter was lower in the developing chicken pallium at all stages examined ( Fig. 5c ). These data suggest that canonical Notch signalling is activated in stage-dependent and species-specific manners in cortical/pallial neural stem/progenitor cells. 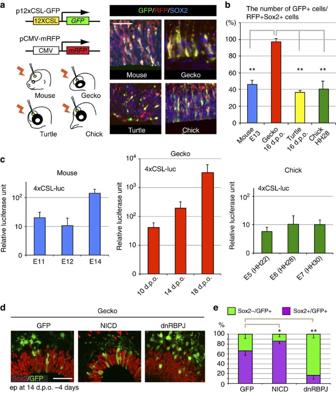Figure 5: Inter-species differences in the activation of Notch signalling in cortical/pallial neural stem/progenitor cells. (a) The expression of an RBPJ-dependent GFP reporter (p12xCSL-GFP) in the developing mouse (E13.5), gecko (16 d.p.o.), turtle (16 d.p.o.) and chicken (HH26) cortices/pallia. Electroporated cells were monitored by the co-electroporation of an RFP expression vector. (b) The proportion of GFP reporter-expressing cells among RFP and Sox2-expressing ventricular cells in distinct amniotes. Values represent mean (n=3 animals in mouse, geckoes and chicken, andn=2 animals in turtles). **P<0.01 (mice, geckos, turtles and chickens: unpaired Student’st-test). (c) Promoter activities of a Notch reporter (p4xCSL-luciferase) in the mouse, gecko and chicken cortices/pallia at various embryonic stages. Values represent mean (n=3 or 4 samples in each stage) and s.d. (d,e) Manipulation of Notch signalling in the developing gecko cortex. Overexpression of NICD or dnRBPJ significantly decreased or increased neuronal differentiation, respectively. Values represent mean (n=3 animals) and s.d. *P<0.05, **P<0.01 (unpaired Student’st-test). Scale bars, 50 μm (a,d). Figure 5: Inter-species differences in the activation of Notch signalling in cortical/pallial neural stem/progenitor cells. ( a ) The expression of an RBPJ-dependent GFP reporter (p12xCSL-GFP) in the developing mouse (E13.5), gecko (16 d.p.o. ), turtle (16 d.p.o.) and chicken (HH26) cortices/pallia. Electroporated cells were monitored by the co-electroporation of an RFP expression vector. ( b ) The proportion of GFP reporter-expressing cells among RFP and Sox2-expressing ventricular cells in distinct amniotes. Values represent mean ( n =3 animals in mouse, geckoes and chicken, and n =2 animals in turtles). ** P <0.01 (mice, geckos, turtles and chickens: unpaired Student’s t -test). ( c ) Promoter activities of a Notch reporter (p4xCSL-luciferase) in the mouse, gecko and chicken cortices/pallia at various embryonic stages. Values represent mean ( n =3 or 4 samples in each stage) and s.d. ( d , e ) Manipulation of Notch signalling in the developing gecko cortex. Overexpression of NICD or dnRBPJ significantly decreased or increased neuronal differentiation, respectively. Values represent mean ( n =3 animals) and s.d. * P <0.05, ** P <0.01 (unpaired Student’s t -test). Scale bars, 50 μm ( a , d ). Full size image To address whether Notch signalling is required for the maintenance of neural stem/progenitor cells in the developing gecko cortex, we performed gain- and loss-of-function analyses of Notch signalling using expression vectors for NICD and the dominant-negative form of RBP-Jk (dnRBP-Jk). At 4 days after electroporation, differentiated neurons and neural stem/progenitor cells were quantified on the basis of Sox2 expression. Compared with controls that were electroporated with the GFP expression vector, NICD-overexpression embryos had a significantly reduced number of differentiated neurons (Sox2-negative GFP-labelled cells: 33.9±9.2% in control embryos, n =3 animals; 14±5.4% in NICD-overexpressing embryos, n =3, Fig. 5d,e ), which indicates that sustaining Notch signalling suppressed neurogenesis in the developing gecko cortex. In contrast, the introduction of the dnRBP-Jk expression vector dramatically enhanced neuronal differentiation (83.4±7.6%, n =3) and decreased the proportion of neural stem/progenitor cells ( Fig. 5d,e ), which indicates that the inhibition of endogenous Notch signalling is sufficient to induce abundant neurogenesis in the gecko cortex. Together, these results indicate that inter-species variation in canonical Notch signalling activity is a central factor in determining the differential neurogenic potentials observed during cortical/pallial development in various amniotes. Sequential generation of neuronal subtypes in geckoes Finally, to address the relationship between the lower rate of neurogenesis and the extent of neuronal diversity in the gecko cortex, we examined the molecular characteristics of gecko cortical neurons. In the mammalian neocortex, several transcription factors are expressed in a lamina-specific manner. Among these factors, CTIP2 is predominantly expressed by layer V projection neurons, whereas SATB2 is detected in the neurons of cortical layer II–IV and VI neurons [33] , [34] ( Supplementary Fig. S6 ). We found that CTIP2 and SATB2 were strongly expressed in the gecko DCx ( Fig. 6 ). In contrast to the mouse cortex, neuronal subtypes expressing CTIP2 or SATB2 were not aligned as radially oriented layers in the gecko cortex: CTIP2-positive cells were distributed at the antero-medial part of the DCx, whereas SATB2-positive cells were detected at the posterior-lateral part of the DCx, although these neuronal populations were significantly intermingled ( Fig. 6a–c,e–g ). In addition, there was a subpopulation of cells in the DCx that expressed both CTIP2 and SATB2 ( Fig. 6c,g ). The expression of Tbr1 and FoxP2, which are the markers for cortical layer VI, were also detected in the developing gecko cortex ( Supplementary Fig. S6 ). CTIP2 and SATB2 were also expressed in the turtle cortex, which suggests that the cortex in reptiles commonly consists of multiple neuronal subtypes distinguished by lamina-specific layer markers ( Fig. 6d,h ). 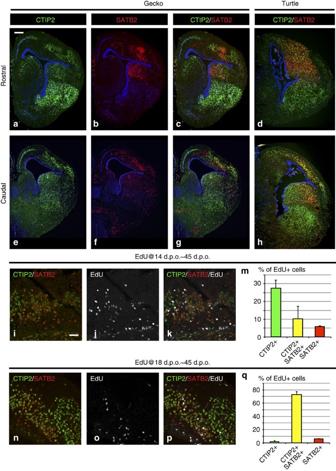Figure 6: Sequential generation of different neuronal subtypes in the developing gecko cortex. (a–h) The distribution of CTIP2- and SATB2-positive cells in the developing cortex of thePictusgecko (a–c,e–g; 44 d.p.o.) and the Chinese soft-shelled turtle cortex (d,h, st25). In the rostral cortex, CTIP2- and SATB2-expressing cells are distributed in a medio-lateral array, whereas in the caudal cortex these neuronal subtypes are intermingled. A similar trend was observed in the turtle cortex. (i–q) Birth dating analyses of different neuronal subtypes in the developing gecko cortex. EdU administration at 14 or 18 d.p.o. labelled distinct neuronal populations. CTIP2 single-positive cells are predominantly born at 14 d.p.o., whereas CTIP2/SATB2 double-positive cells and SATB2 single-positive cells are at both 14 and 18 d.p.o. (m,q). Values represent mean (n=2 animals) and range. Scale bars, 200 μm (a), 50 μm (i). Figure 6: Sequential generation of different neuronal subtypes in the developing gecko cortex. ( a – h ) The distribution of CTIP2- and SATB2-positive cells in the developing cortex of the Pictus gecko ( a – c , e – g ; 44 d.p.o.) and the Chinese soft-shelled turtle cortex ( d , h , st25). In the rostral cortex, CTIP2- and SATB2-expressing cells are distributed in a medio-lateral array, whereas in the caudal cortex these neuronal subtypes are intermingled. A similar trend was observed in the turtle cortex. ( i – q ) Birth dating analyses of different neuronal subtypes in the developing gecko cortex. EdU administration at 14 or 18 d.p.o. labelled distinct neuronal populations. CTIP2 single-positive cells are predominantly born at 14 d.p.o., whereas CTIP2/SATB2 double-positive cells and SATB2 single-positive cells are at both 14 and 18 d.p.o. ( m , q ). Values represent mean ( n =2 animals) and range. Scale bars, 200 μm ( a ), 50 μm ( i ). Full size image In mammalian corticogenesis, lamina-specific neurons are successively generated in a temporally ordered manner. To examine whether a temporal pattern of neuronal subtype specification exists in the gecko cortex, we performed birth date analyses of CTIP2 and/or SATB2-positive cortical neurons by administrating small amounts of EdU into the developing brain vesicles. We injected EdU at 14 or 18 d.p.o., and examined the expression of lamina-specific markers in EdU-labelled cells at 37–45 d.p.o. Pulse labelling of neurons born at different developmental stages indicated the successful generation of specific neuronal subtypes in the gecko DCx. Neurons labelled with EdU at 14 d.p.o. predominantly expressed only CTIP2, whereas those labelled with EdU exposure at 18 d.p.o. predominantly expressed both CTIP2 and SATB2 ( Fig. 6i–q ). Notably, equal proportions of SATB2-positive neurons were observed in embryos labelled with EdU at 14 or 18 d.p.o., which suggests that this type of neurons is continuously generated during the neurogenic period ( Fig. 6m,q ). These results indicate that the temporal specification mechanisms that generate laminar neuronal subtypes are evident in the cortex of reptiles, although the proliferation and differentiation capacities of neural stem/progenitor cells are significantly lower in reptiles than in mammals. Changes in developmental mechanisms governing cell proliferation and differentiation are thought to have critical roles in the evolutionary expansion of the brain [35] . Here, we determined that the frequencies of cell division in the gecko cortex are significantly lower than those observed in other amniotes. This difference is primarily the result of a long cell-cycle length and the prevalence of self-renewing of neural stem/progenitor cells in the gecko. As neurogenesis in the gecko cortex terminates at the early embryonic stages, total rounds of cell division during the cortical neurogenic period might be limited. Furthermore, proliferating basal progenitors, which are responsible for an extensive increase of neuron numbers in the mammalian cortex [36] , are missing in the gecko cortex. Thus, the relatively inactive character of gecko cortical ventricular cells provides less amplification of the progenitor pool and of neurons, which may contribute to a minimum elaboration of the DCx in this species. The number of apical mitotic cells in the gecko pallium exhibited a medial-low and lateral-high gradient, as seen in the mouse pallium. A similar pattern of proliferation kinetics has been reported in the developing avian pallium [13] , [37] . These data suggest that the common regulatory mechanisms govern spatial differences in progenitor divisions across amniote species. Aboitiz [38] suggested that the upregulation of Pax6 provided the expansion of the ventral pallium in non-mammalian amniotes and that the additional enhancement of dorsal factors, such as Wnt signalling, contributed to massive elaboration of the dorsal pallium in the mammalian lineage. Of note, the secondary proliferative zone is also observed in the avian ventral pallium [39] , which resembles the mammalian cortical SVZ. As we could not detect such a proliferative zone in the gecko pallium, the secondary proliferative zone might have evolved independently in the mammalian and arcosaurian lineages but by recruiting similar regulatory mechanisms. Luzzati et al. [40] hypothesized that the regulatory mechanisms for making the mammalian dorsal pallium may have been co-opted from those in the reptilian ventral pallium. Recent studies have elucidated the genetic mechanisms underlying cell division frequencies and cell-cycle length during murine cortical development [41] , [42] , which provides insights into the regulation of the species-specific proliferation kinetics of cortical neural stem/progenitor cells. We showed that Notch signalling is highly activated in the developing gecko ventricular cells, which significantly constrains the frequency of neuronal differentiation. Consistently, the constitutive activation of Notch-signalling components suppresses neuronal differentiation in various vertebrate species [43] , [44] , [45] . Furthermore, there are remarkable differences in the Notch activation status in the cortical neural stem/progenitor cells of amniotes. Therefore, the spatio-temporal regulation of Notch signalling in neural stem/progenitor cells may provide a molecular basis for the inter-species differences in pallial neurogenic rates. In the developing mouse brains, the mosaic activation of Notch signalling in the neural stem/progenitor cells is essential for cell-cycle progression and neuronal differentiation [32] , [43] . It is noteworthy that turtles and chickens also exhibit mosaic patterns of Notch activation and rapid neuronal outputs during corticogenesis. Recent genomic analysis revealed that turtles are included in the archosaurs as a sister group of birds [46] , [47] . Thus, our data provide the first evidence that turtles and birds share developmental characteristics with respect to cortical neurogenesis. Despite minimal rates of neurogenesis, our results, together with recent findings by others [48] (including Drs I.K. Suzuki and T. Hirata, personal communication), indicate that the reptilian cortex possesses distinct neuronal subtypes distinguished by the expression of specific transcription factors. Furthermore, we revealed the successive generation of neuronal subtypes in the developing gecko cortex, similar to the mammalian cortex and avian pallium. Previous studies reported that the reptilian trilaminar cortex lacks neurons homologous to the mammalian superficial layer neurons and that these neuronal subtypes are an evolutionary innovation in the mammalian lineage [17] , [18] . Currently, we do not have enough evidence concerning the existence of a homologue of mammalian superficial layer neurons in the reptilian cortex. Nevertheless, our data strongly suggest that all amniotes share the developmental programme for temporally ordered neuron subtype specification in the dorsal part of the telencephalon. These lines of evidence provide a possible scenario for the multiple evolutionary steps towards convergent encephalization in amniotes ( Fig. 7 ). First, a temporally ordered neurogenic programme has been acquired in the basal amniotes, and the modification of this programme results in the elaboration of lineage-specific cortical/pallial architectures. Interestingly, distinct neuronal subtypes are spatially distributed in the gecko DCx, as in the chicken pallium [12] , [13] . This similarity suggests that temporally organized neurogenic programme in mammalian lineages had evolved by the re-organization of spatially segregated neurogenic programmes. However, Suzuki et al. [13] also clarified that avian pallial neural progenitors have a potential to produce multiple neuronal subtypes sequentially in dissociated culture condition. This finding suggests that the temporally regulated neurogenic system is the ‘default’ status that is derived from a common ancestor(s) of amniotes. The spatial regulation of neurogenesis in chicken is attributed to different proliferation kinetics, which might be governed by local signalling molecules in the developing telencephalon [13] , [38] . 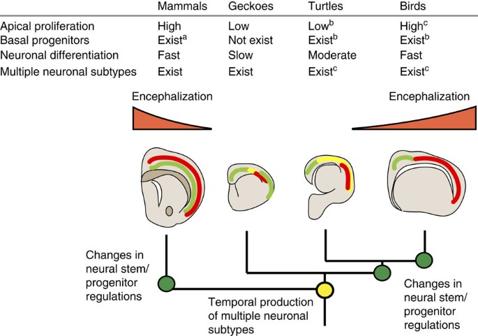Figure 7: A schematic diagram showing a possible scenario of cortical evolution. We hypothesized that parallel encephalization had occurred independently in distinct amniote lineages through changes in cortical neural stem/progenitor dynamics. Modification of Notch signalling activity may have contirubuted to the acceleration of neuronal differentiation, and simultaneous and/or subsequent changes in developmental programmes may have resulted in enhanced proliferation in the ventricular zone and the emergence of basal progenitors in the subventricular zone.aBasal progenitors are only recognized in eutherian mammals49.bLower proliferation of apical progenitors in turtles, and the existence of abventricular mitotic cells in turtles and birds have been reported39. In contrast, the temporal generation of multiple neuoronal subtypes may have been acquired by a common ancestor(s) of amniotes.cA high proliferation activity of apical progenitors and the exsistence of multiple neuronal subtypes in the avian pallium have been reported12,13,48. Figure 7: A schematic diagram showing a possible scenario of cortical evolution. We hypothesized that parallel encephalization had occurred independently in distinct amniote lineages through changes in cortical neural stem/progenitor dynamics. Modification of Notch signalling activity may have contirubuted to the acceleration of neuronal differentiation, and simultaneous and/or subsequent changes in developmental programmes may have resulted in enhanced proliferation in the ventricular zone and the emergence of basal progenitors in the subventricular zone. a Basal progenitors are only recognized in eutherian mammals [49] . b Lower proliferation of apical progenitors in turtles, and the existence of abventricular mitotic cells in turtles and birds have been reported [39] . In contrast, the temporal generation of multiple neuoronal subtypes may have been acquired by a common ancestor(s) of amniotes. c A high proliferation activity of apical progenitors and the exsistence of multiple neuronal subtypes in the avian pallium have been reported [12] , [13] , [48] . Full size image We also hypothesized that changes in the regulation of neural stem/progenitor cells, including the activation mechanisms of Notch signalling, occurred in the ancestors of mammals and archosaurs independently. Further changes in the proliferation of apical progenitors and the emergence of basal progenitors might have contributed to the massive neurogenesis and expansion of the cerebrum in the mammalian and avian lineages. Although we could not eliminate the possibility that unique characteristics of gecko corticogenesis have been acquired secondarily, recent reports support the convergent evolution of basal progenitors (abventricular mitotic cells) in distinct lineages of amniotes [39] , [49] . As a six-layered laminar structure in extant mammals and massive elaboration of dorsal ventricular ridge in birds are highly apomorphic brain traits [50] , analyses of reptilian cortical development will provide further clues to understanding the changes in the molecular mechanisms underlying the distinct styles of amniote pallial architectures. Animals Adult Madagascar ground geckos ( P. pictus, four males and four females) were obtained from Kansai Reptile Pro (Osaka, Japan), and maintained in our laboratory (14 h: 10-h light–dark cycles at 28 °C). After breeding, each female laid two eggs every 7–10 days for several months, and a total of 192 eggs were oviposited by four females. Fertilized eggs were collected and incubated at 28 °C in an incubator until the stages of interest. Developmental stages in the geckos were determined according to a previous report [19] . Fertilized eggs of Chinese soft-shelled turtles were obtained from a local breeder (Daiwa Yoshoku, Saga, Japan), and incubated at 28 °C. Developmental stages were determined according to a previous report [51] . Fertilized chicken eggs were obtained from a local poultry farm (Yamagishi Farm, Japan) and incubated at 37 °C. Pregnant female mice (CD-1 background, 3 months) were purchased from Japan Charles River Inc. All animal experiments were approved by the Committee of the Kyoto Prefectural University of Medicine. Immunohistochemistry Brains were fixed with 4% paraformaldehyde dissolved in PBS at 4 °C for overnight. After washing with PBS, the brains were cryoprotected with 30% sucrose solution and immersed in Tissue-Tek. Frozen brains were sectioned at a thickness of 14–16 μm using a Cryostat (Leica CM1900 and CM1850, Germany), and incubated with primary antibodies, including anti-Sox2 (rabbit polyclonal, Abcam), anti-ßIII tubulin (1:100, mouse monoclonal, Millipore), anti-phosphorylated histone H3 (1:200, rabbit polyclonal, Millipore), anti-Tbr2 (1:500, rabbit polyclonal, Abcam), anti-PAX6 (1:500, mouse monoclonal, Developmental Studies Hybridoma Bank), anti-GFP (1:500, rabbit polyclonal, Life Technologies or rat monoclonal, Nakarai Tesque), anti-RFP (1:500, rabbit polyclonal, Abcam), anti-RBP-Jk (1:2,000, rat monoclonal, Cosmo Bio), anti-CTIP2 (1:500, rat monoclonal, Abcam), anti-SATB2 (1:200, mouse monoclonal, Abcam), anti-Tbr1 (1:200, chicken polyclonal, Millipore) and anti-FoxP2 (1:500, rabbit polyclonal, Abcam) antibodies. After washing, sections were incubated with secondary antibodies, including Alexa-Fluor 488, 594 or 633-conjugated anti-rabbit, anti-mouse and anti-rat antibodies (1:500, Life Technologies). For extensive amplification of signals, the sections were incubated with biotinylated anti-rat or anti-rabbit antibodies, processed with the Vectastain ABC Kit (Vector Laboratory) and treated with the Tyramide Signal Amplification System (TSA system; PerkinElmer). The sections were analysed with either a fluorescent microscope (BX51, Olympus) equipped with a cooled CCD system (DP71, Olympus) or with a laser confocal microscope (FV1000D, Olympus). Determination of cell-cycle length Cell-cycle length was determined by the sequential administration of the distinct thymidine analogus, EdU and BrdU. First, 0.1 μl of EdU solution (10 mg ml −1 ) was injected into the Pictus brain ventricle. After 1.5 h, the same amount of BrdU solution (10 mg ml −1 ) was injected into the brain ventricle and incubated for 30 min before fixation. EdU was detected by the Click-iT EdU Detection System (Life Technologies), followed by immunostaining with several antibodies. To detect BrdU-labelled cells, the sections were post-fixed with 4% PFA for 30 min before being treated with 2 N HCl at 37 °C for 15 min (denaturation) and incubated with an anti-BrdU antibody (Life Technologies) that specifically recognizes BrdU but not EdU. Luciferase reporter assay p4xCSL-firefly luciferase [52] , pCAGGS-Renilla luciferase and pCAGGS-GFP vectors were co-electroporated into the developing mouse, gecko and chicken cortices/palllia at various embryonic stages. Owing to the limited accessibility and high mortality of embryos, early stages of mouse embryos (E10) and all stages of gecko embryos were electroporated and cultured in the whole-embryo culture system (Ikemoto Rika Kogyo; supplied with 95% oxygen and kept at 37 °C for mice and 30 °C for geckos). After 1 or 2 days of in utero/ex utero / in ovo electroporation, cortical/pallial tissues containing GFP-positive cells were dissected out under a fluorescent microscope, and Notch reporter activity was examined with the dual-luciferase reporter assay system (Promega). Chemical luminescence was analysed with a micro-plate reader (2030 ARVO X , PerkinElmer). All of firefly luciferase values were normalized with reference to Renilla luciferase activities and multiplied by 10 6 to establish relative luciferase units. In ovo electroporation In ovo electroporation of the developing gecko, turtle, and chicken embryo was performed according to the method for quail embryos [12] . Briefly, after cleaning the surface of the egg, a small window was opened in the shell using fine forceps, and ~0.1 μl of DNA solution was injected into the lateral ventricle using a small glass needle. Needle-type electrodes (CUY200S, Neppa Gene, Japan) were placed close to the injected area of the brain, and square pulses (30 V, 50 ms, twice) were applied with an electric stimulator (Nihon Koden, Japan). After electroporation, the extraembryonic cavity was filled with sterilized PBS containing antibiotics (Gentamycin or Penicillin/Streptomycin), and the window was sealed with a round cover glass to prevent drying out and microbe contamination. Operated embryos were incubated at 28 °C under high humidity until the necessary stages. To prepare the DNA solution, various expression vectors including pCAX-GFP, pCAGGS-mRFP (a gift from Dr Uchikawa), pCIG-Cre, pCMV-Brainbow1.0L (obtained from Addgene: ID18721), p12xCSL-GFP, p4xCSL-firefly luciferase (obtained from Addgene: ID41726), pCAGGS-Renilla luciferase (a gift from Dr De Pietri Tonelli), pNICD and pFuggie-dnRBPJ-ires-GFP were dissolved in PBS (2.5–5 μg μl −1 ) containing 0.05% of Fast green. In utero electroporation In utero electroporation of mouse embryos was performed with slight modification of previous methods [53] , [54] . Pregnant female mouse was anesthetized by intraperinoneally injection of avertin, and incision was made in the abdominal wall to expose uterus horn. DNA solution was injected into the lateral ventricle of embryos, and square pulses (35 V, 50 ms, four times) were applied to the embryos with a tweezer-type electrode (CUY650P3) connected with the electric stimulator (Nihon Koden). How to cite this article: Nomura, T. et al. Changes in the regulation of cortical neurogenesis contribute to encephalization during amniote brain evolution. Nat. Commun. 4:2206 doi: 10.1038/ncomms3206 (2013).